OTUB1 enhances TGFβ signalling by inhibiting the ubiquitylation and degradation of active SMAD2/3 SMAD transcription factors are key intracellular transducers of TGFβ cytokines. SMADs are tightly regulated to ensure balanced cellular responses to TGFβ signals. Ubiquitylation has a key role in regulating SMAD stability and activity. Several E3 ubiquitin ligases that regulate the turnover of SMADs are known; however, proteins that prevent the ubiquitylation or cause deubiquitylation of active SMADs remain undefined. Here we demonstrate that OTUB1 is recruited to the active phospho-SMAD2/3 complex only on TGFβ induction. Further, OTUB1 has a crucial role in TGFβ-mediated gene transcription and cellular migration. OTUB1 inhibits the ubiquitylation of phospho-SMAD2/3 by binding to and inhibiting the E2 ubiquitin-conjugating enzymes independent of its catalytic activity. Consequently, depletion of OTUB1 in cells causes a rapid loss in levels of TGFβ-induced phospho-SMAD2/3, which is rescued by the proteasomal inhibitor bortezomib. Our findings uncover a signal-induced phosphorylation-dependent recruitment of OTUB1 to its target in the TGFβ pathway. The signalling pathways triggered by the transforming growth factor-β (TGFβ) family of cytokines control a plethora of cellular functions during embryogenesis and in adult tissues, including differentiation, proliferation, survival, extracellular matrix production and migration. Consequently, abnormal TGFβ signalling is associated with multiple human diseases such as fibrosis, immune disorders and cancer [1] , [2] , [3] , [4] . TGFβ signalling is initiated on ligand binding to a pair of receptor serine/threonine protein kinases (termed type II and type I) on the cell surface. This triggers the phosphorylation of receptor-regulated SMAD transcription factors (R-SMADs) at their conserved C-terminal SXS motif (tail phosphorylation) by the type I receptors [5] . TGFβ ligands are divided into two subfamilies. The TGFβ subfamily primarily signals through the phosphorylation of SMADs 2 and 3, whereas the bone morphogenetic protein (BMP) subfamily signals through SMADs 1/5/8 (ref. 5 ). Once phosphorylated, R-SMADs interact with SMAD4 and translocate to the nucleus, where together with other cofactors, they regulate the transcription of over 500 target genes [5] , [6] , [7] . Complex mechanisms, which are often context dependent, have evolved to check and modulate the potent activity of TGFβ ligands in controlling cell behaviour and tissue homoeostasis [8] , [9] . Although the regulation of the TGFβ pathway occurs at multiple layers of the signalling cascade, R-SMADs, as critical mediators of TGFβ signals, are suitably primed for key regulatory inputs. Indeed, reversible phosphorylation and ubiquitylation of SMAD proteins are critical processes that regulate the potency and duration of TGFβ signalling [10] , [11] . The mechanisms of ubiquitin-mediated turnover of R-SMADs by distinct E3 ubiquitin ligases are generally well established [10] , [12] , [13] , [14] , [15] , [16] . In particular, phosphorylation of the linker region of R-SMADs by CDK8/9, mitogen-activated protein kinases and GSK-3 marks R-SMADs for recognition by E3 ubiquitin ligases SMURF1/NEDD4L, which mediate their polyubiquitylation and degradation [14] , [16] , [17] . On the other hand, the turnover of active SMADs is likely to be regulated either by removal of the polyubiquitin chains by selective deubiquitylating enzymes (DUBs) or prevention of polyubiquitylation to produce a dynamic fine-tuning of signalling. In the TGFβ pathway, candidate proteins that recognize active SMADs and either deubiquitylate or prevent their ubiquitylation remain elusive. A proteomic screen undertaken to identify novel interactors of R-SMADs isolated OTUB1 (OTU domain, ubiquitin aldehyde binding 1) in green fluorescent protein (GFP)-SMAD3 immunoprecipitates only from cells treated with TGFβ. OTUB1 belongs to the ovarian tumour domain protease (OTU) family of DUBs that comprises 14 other members [18] . The canonical mode of action for OTUB1 to function is as a cysteine protease that hydrolyses the isopeptide bond between ubiquitin and the target or another ubiquitin molecule. The catalytic triad of OTUB1 is composed of D88/C91/H265 in the OTU domain, and a ubiquitin-binding motif is present in the N terminus [19] , [20] , [21] , [22] . OTUB1 has been reported to deubiquitylate TRAF3/6 (ref. 23 ), oestrogen receptor-α (ref. 24 ), p53 (ref. 25 ), c-IAP1 (ref. 26 ) and act as a specific receptor for ubiquitylated GRAIL [27] and stabilize active RhoA [28] . Recently, several studies have described a non-canonical mode of OTUB1 action in which OTUB1 inhibits the ubiquitylation of target proteins by binding to and inhibiting the E2 ubiquitin-conjugating enzyme UBE2N (also known as UBC13) independent of its catalytic activity [29] , [30] , [31] , [32] . In the present study, we identify OTUB1 as a novel component of the TGFβ-induced active R-SMAD complex and demonstrate that it is essential for TGFβ-induced gene transcription and cellular migration. We propose that the ability of OTUB1 to interact with SMAD2/3 and inhibit their polyubiquitylation, independent of catalytic activity, is necessary and sufficient for the regulation of TGFβ signalling. Further, our study uncovers a signal-induced phosphorylation-dependent recruitment of OTUB1 to its target in the TGFβ pathway. Identification of OTUB1 as an interactor of GFP-SMAD3 To uncover novel modes of regulation of the TGFβ pathway, we employed a proteomic approach to identify interactors of SMAD3, a key mediator of the TGFβ ligands. As a control, we used SMAD1, a mediator of the BMP signals. Human Embryonic Kidney 293 (HEK293) cells stably expressing N-terminally GFP-tagged SMAD1 or SMAD3 under the control of a tetracycline inducible promoter were generated as described previously [33] . GFP immunoprecipitates (IPs) were resolved by SDS-polyacrylamide gel electrophoresis (PAGE) and the interacting proteins were excised, digested with trypsin and identified by mass spectrometry ( Fig. 1a ). As expected, BMP and TGFβ treatment resulted in the phosphorylation of GFP-SMAD1 and GFP-SMAD3, respectively ( Supplementary Fig. S1a ). Previously reported R-SMAD interactors, including SMAD4, LEMD3, TRIM33 and SKI were identified in GFP-SMAD1 and GFP-SMAD3 IPs as indicated ( Fig. 1a ) [34] , [35] , [36] , [37] , [38] , [39] . OTUB1 was identified as a novel interactor of GFP-SMAD3 only when cells were treated with TGFβ ( Fig. 1a ). Four OTUB1 tryptic peptides were identified representing 8% sequence coverage ( Fig. 1a ). OTUB1 is ubiquitously expressed in mouse tissues ( Supplementary Fig. S1b ) and across many human cell lines, with relatively high expressions observed in breast cancer cells ( Supplementary Fig. S1c ). 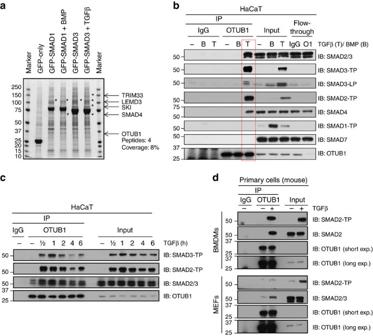Figure 1: OTUB1 interacts with TGFβ-stimulated SMAD2/3/4. (a) HEK293 cells stably expressing GFP-only, GFP-SMAD1 or GFP-SMAD3 were treated with 50 pM TGFβ or 25 ng ml−1BMP for 1 h before lysis in the presence of dithiobis[succinimidyl propionate] (DSP). GFP immunoprecipitates (IPs) were separated by SDS-PAGE and interacting partners identified by mass spectrometry. (b) An endogenous IP with OTUB1 antibody or pre-immune sheep IgG was performed in HaCaT cell extracts, stimulated without or with 50 pM TGFβ or 25 ng ml−1BMP for 1 h. Cell extracts (input), endogenous IgG or OTUB1 IPs and the corresponding immune-depleted flow-through extracts (O1=OTUB1-depleted untreated HaCaT extract) were resolved by SDS-PAGE and immunoblotted (IB) with the indicated antibodies. (c) As inb, except that a time course of 50 pM TGFβ treatment was performed for up to 6 h before lysis. (d) An endogenous IP with anti-OTUB1 antibody or pre-immune sheep IgG was performed in extracts from bone marrow-derived macrophages (BMDMs) and mouse embryonic fibroblasts (MEFs) stimulated with or without 50 pM TGFβ for 1 h. Before TGFβ stimulation, BMDMs were serum starved for 2 h, whereas MEFs were not starved. Cell extracts (input) or IPs were resolved by SDS-PAGE and immunoblotted with the indicated antibodies. SMAD-LP, linker-phosphorylated SMAD; SMAD-TP, tail-phosphorylated SMAD. Figure 1: OTUB1 interacts with TGFβ-stimulated SMAD2/3/4. ( a ) HEK293 cells stably expressing GFP-only, GFP-SMAD1 or GFP-SMAD3 were treated with 50 pM TGFβ or 25 ng ml −1 BMP for 1 h before lysis in the presence of dithiobis[succinimidyl propionate] (DSP). GFP immunoprecipitates (IPs) were separated by SDS-PAGE and interacting partners identified by mass spectrometry. ( b ) An endogenous IP with OTUB1 antibody or pre-immune sheep IgG was performed in HaCaT cell extracts, stimulated without or with 50 pM TGFβ or 25 ng ml −1 BMP for 1 h. Cell extracts (input), endogenous IgG or OTUB1 IPs and the corresponding immune-depleted flow-through extracts (O1=OTUB1-depleted untreated HaCaT extract) were resolved by SDS-PAGE and immunoblotted (IB) with the indicated antibodies. ( c ) As in b , except that a time course of 50 pM TGFβ treatment was performed for up to 6 h before lysis. ( d ) An endogenous IP with anti-OTUB1 antibody or pre-immune sheep IgG was performed in extracts from bone marrow-derived macrophages (BMDMs) and mouse embryonic fibroblasts (MEFs) stimulated with or without 50 pM TGFβ for 1 h. Before TGFβ stimulation, BMDMs were serum starved for 2 h, whereas MEFs were not starved. Cell extracts (input) or IPs were resolved by SDS-PAGE and immunoblotted with the indicated antibodies. SMAD-LP, linker-phosphorylated SMAD; SMAD-TP, tail-phosphorylated SMAD. Full size image OTUB1 interacts with the active SMAD2/3/4 complex To verify the ligand inducible interaction between OTUB1 and SMAD3 at the endogenous level, OTUB1 was immunoprecipitated from human keratinocyte HaCaT cell extracts. OTUB1 was efficiently immunoprecipitated with the anti-OTUB1 antibody but not with pre-immune IgG ( Fig. 1b ). TGFβ induces formation of the active phospho-SMAD2/3-SMAD4 transcription complex [34] , [35] . Tail (TP)- and linker (LP)-phosphorylated SMAD3, total SMAD3, SMAD2-TP and total SMAD2 were all detected in OTUB1 IPs from cells stimulated with TGFβ but not from BMP or unstimulated controls ( Fig. 1b ). SMAD4 was also detected in OTUB1 IPs only on TGFβ stimulation ( Fig. 1b ), indicating that OTUB1 binds to the active SMAD2/3/4 complex. Endogenous SMAD1-TP and SMAD4 were not detected in OTUB1 IPs from control or BMP-treated extracts ( Fig. 1b ), suggesting that OTUB1 selectively recognizes the TGFβ-induced SMAD complexes. SMAD7, a transcriptional target of both BMP and TGFβ signalling, was also not detected in OTUB1 IPs ( Fig. 1b ). None of the SMADs were detected in pre-immune sheep IgG IPs, employed as control ( Fig. 1b ). We also investigated the kinetics of OTUB1–SMAD2/3 interaction on TGFβ stimulation in HaCaT cells. The binding of endogenous OTUB1 to the active SMAD2/3/4 complex occurred within 30 min of TGFβ stimulation and persisted through 6 h of continuous stimulation, closely mirroring the levels of SMAD2/3 tail phosphorylation ( Fig. 1c ). The TGFβ-induced interaction between OTUB1 and SMAD2/3 was also confirmed in primary cells derived from mice ( Fig. 1d ). SMAD2-TP and total SMAD2 were detected in OTUB1 IPs from primary bone marrow-derived macrophages (BMDMs) and mouse embryonic fibroblasts (MEFs) only when cells were treated with TGFβ ( Fig. 1d ). Phosphorylation of SMAD2/3 is necessary for OTUB1 binding As shown in Fig. 1 , OTUB1 selectively binds components of the active phospho-SMAD2/3-SMAD4 complex; however, it was not clear whether SMAD4 was required for this interaction. Therefore, we employed the SW480 colon cancer cell line, which lacks SMAD4 expression [40] . In both HaCaT and SW480 cells, TGFβ induced the phosphorylation of SMAD2/3 ( Fig. 2a ). In both cells, phospho-SMAD2/3 proteins were detected in OTUB1 IPs on TGFβ stimulation ( Fig. 2a ). SW480 cells displayed elevated basal levels of phospho-SMAD2/3 over HaCaT cells ( Fig. 2a ). Consistent with this, even in the absence of TGFβ stimulation, phospho-SMAD2/3 were detected in OTUB1 IPs in SW480 cells ( Fig. 2a ). These observations imply that SMAD4 is not required for the interaction between OTUB1 and phospho-SMAD2/3. 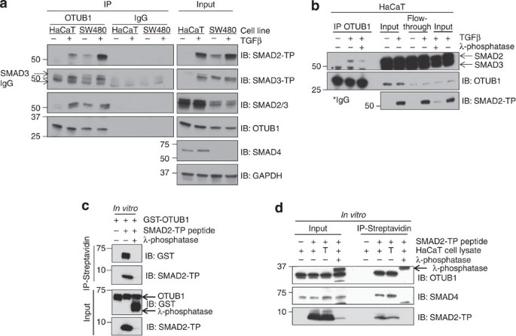Figure 2: OTUB1 binding to SMAD2/3 is phosphorylation dependent. (a) An endogenous IP with OTUB1 antibody or pre-immune sheep IgG was performed in HaCaT and SW480 cell extracts, stimulated with or without 50 pM TGFβ for 1 h before lysis. Extracts (input) and endogenous OTUB1 or IgG IPs were resolved by SDS-PAGE and immunoblotted with the indicated antibodies. (b) Endogenous OTUB1 was immunoprecipitated from HaCaT cells treated with or without TGFβ (50 pM; 1 h) before lysis. After washing, the IPs were then treated with or without lambda (λ) phosphatase for 30 min at 30 °C and washed four times. As a control, an aliquot of TGFβ-treated cell extract was incubated with λ-phosphatase for 30 min at 30 °C. Cell extracts, IPs and flow-throughs were resolved by SDS-PAGE and immunoblotted with the indicated antibodies. (c) Purified GST-OTUB1 was incubated with biotin-tagged phospho-SMAD2 peptide in the presence or absence of λ-phosphatase for 30 min at 30 °C. The SMAD2 peptide was immunoprecipitated with streptavidin beads and washed six times. Input and IP samples were resolved by SDS-PAGE and immunoblotted with the indicated antibodies. (d) As inc, however, the SMAD2 peptide was incubated with untreated HaCaT (+) or TGFβ (T; 50 pM; 1 h)-treated cell lysate. SMAD4 antibody is used as a positive control. Figure 2: OTUB1 binding to SMAD2/3 is phosphorylation dependent. ( a ) An endogenous IP with OTUB1 antibody or pre-immune sheep IgG was performed in HaCaT and SW480 cell extracts, stimulated with or without 50 pM TGFβ for 1 h before lysis. Extracts (input) and endogenous OTUB1 or IgG IPs were resolved by SDS-PAGE and immunoblotted with the indicated antibodies. ( b ) Endogenous OTUB1 was immunoprecipitated from HaCaT cells treated with or without TGFβ (50 pM; 1 h) before lysis. After washing, the IPs were then treated with or without lambda (λ) phosphatase for 30 min at 30 °C and washed four times. As a control, an aliquot of TGFβ-treated cell extract was incubated with λ-phosphatase for 30 min at 30 °C. Cell extracts, IPs and flow-throughs were resolved by SDS-PAGE and immunoblotted with the indicated antibodies. ( c ) Purified GST-OTUB1 was incubated with biotin-tagged phospho-SMAD2 peptide in the presence or absence of λ-phosphatase for 30 min at 30 °C. The SMAD2 peptide was immunoprecipitated with streptavidin beads and washed six times. Input and IP samples were resolved by SDS-PAGE and immunoblotted with the indicated antibodies. ( d ) As in c , however, the SMAD2 peptide was incubated with untreated HaCaT (+) or TGFβ (T; 50 pM; 1 h)-treated cell lysate. SMAD4 antibody is used as a positive control. Full size image To establish whether the phosphorylation of SMAD2/3 in response to TGFβ is critical for its interaction with OTUB1, we λ-phosphatase-treated OTUB1 IPs from TGFβ-treated HaCaT extracts ( Fig. 2b ). This resulted in a significant dissociation of SMAD2 from OTUB1 IPs indicating that phosphorylation of SMAD2 in response to TGFβ is necessary for its interaction with OTUB1. As expected, λ-phosphatase efficiently dephosphorylated TGFβ-induced phospho-SMAD2 in extracts ( Fig. 2b ; input). Further, endogenous OTUB1 IPs were capable of interacting with wild-type FLAG-SMAD3 and phospho-mimetic mutant of FLAG-SMAD3 but not phospho-deficient mutant of FLAG-SMAD3 overexpressed in U2OS cells ( Supplementary Fig. S1d ). To definitively establish whether the interaction of OTUB1 with SMAD2 is tail phosphorylation dependent, we generated a biotin-tagged SMAD2 tail peptide (incorporating residues 428–467 of hSMAD2) phosphorylated at the S*MS* motif (SMAD2 phospho-peptide). When the SMAD2 phospho-peptide was incubated with purified glutathione S-transferase-tagged (GST-OTUB1) protein in vitro, a robust OTUB1 interaction was observed ( Fig. 2c ; lane 2). This interaction was abolished upon λ-phosphatase treatment to dephosphorylate the SMAD2 phospho-peptide ( Fig. 2c ; lane 3). These observations suggest that the interaction between OTUB1 and phospho-SMAD2 is direct. Further, only SMAD2 phospho-peptide but not the λ-phosphatase-treated phospho-peptide was able to pull down endogenous OTUB1 from HaCaT cell extracts independent of TGFβ treatment ( Fig. 2d ). As expected, SMAD4, which is known to interact with SMAD2-TP [35] , also interacted with SMAD2 phospho-peptide ( Fig. 2d ). OTUB1 enhances TGFβ-mediated gene transcription The ligand inducible interaction between OTUB1 and phospho-SMAD2/3 indicates that OTUB1 could have a regulatory role in the TGFβ pathway. We hypothesized that depleting OTUB1 expression from cells might promote the ubiquitylation of active phospho-SMAD2/3 and thus result in the inhibition of TGFβ signalling. Mouse myoblast C2C12 cells stably integrated with a TGFβ-responsive CAGA-luciferase reporter construct were transfected with multiple short interfering RNAs (siRNAs) targeting Otub1 ( Fig. 3a ). Depletion of Otub1 with iOTUB1# 1, yields >90% knockdown of Otub1 protein levels ( Fig. 3a ) resulting in significant inhibition of TGFβ-induced CAGA-luciferase reporter activity compared with control siRNA (mouse iFoxO4; Fig. 3b ). Similar results were obtained with iOTUB1# 3, which yielded >80% depletion in Otub1 expression ( Fig. 3a and Supplementary Fig. S2 ). These results suggest that Otub1 enhances TGFβ-induced transcriptional responses. To confirm the repression of TGFβ-mediated transcription on OTUB1 depletion, we tested the expression of endogenous TGFβ target genes by quantitative reverse transcription (qRT)-PCR in HaCaT cells ( Fig. 3c ). HaCaT cells were transiently transfected with a control siRNA (human iFoxO4) , human OTUB1#1 siRNA or a stable short hairpin RNA ( shRNA ) against OTUB1. On depletion of OTUB1 by both transient and stable knockdown methods, TGFβ-induced PAI-1 messenger RNA expression was significantly inhibited ( Fig. 3d ). The expression of another TGFβ target gene, CTGF , was also significantly inhibited upon siRNA -mediated depletion of OTUB1 ( Fig. 3e ). 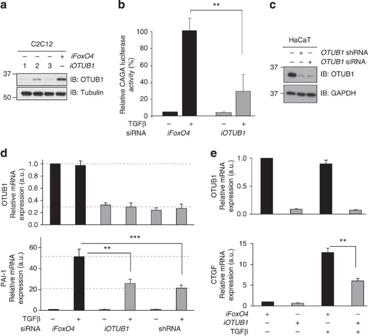Figure 3: Depletion of OTUB1 represses TGFβ-induced transcription. (a) C2C12 cells were transfected with three different siRNAs (#1, #2 and #3) targeting mouse OTUB1 (300 pM/10-cm dish each) and lysed 48 h after transfection. Extracts were resolved by SDS-PAGE and immunoblotted with OTUB1 and tubulin antibodies. (b) C2C12 cells stably expressing a SMAD3-dependent TGFβ-responsive CAGA-luciferase reporter construct were transfected withiFoxO4oriOTUB1#1. Cells were treated with or without 50 pM TGFβ for 6 h before lysis and luciferase activity was measured. Data are represented as mean and error bars indicate s.d. (n=3). (c) HaCaT cells stably expressing shRNA against OTUB1 or transfected with control (−) or OTUB1 siRNA (300 pM/10-cm dish each) for 48 h were lysed, and extracts were resolved by SDS-PAGE and immunoblotted with OTUB1 and GAPDH antibodies. (d) HaCaT cells, transfected with humanOTUB1siRNA, humanFoxO4siRNA, or stably expressing OTUB1 shRNA, were treated with 50 pM TGFβ for 4 h before RNA isolation. Relative expression levels of indicated mRNAs were analysed by qRT-PCR. Data are represented as mean and error bars indicate s.d. (n=6). (e) HaCaT cells depleted of human OTUB1 orFoxO4by RNAi were treated with 50 pM TGFβ for 1 h. TGFβ was then washed off and SB505124 (1 μM) added. RNA was isolated 45 min after TGFβ removal. Relative expression levels of OTUB1 and CTGF mRNAs were analysed by qRT-PCR. Data are represented as mean and error bars indicate s.d. (n=6). Statistical significance of differences between experimental groups was assessed with Student’st-test. **P<0.01 and ***P<0.001. Figure 3: Depletion of OTUB1 represses TGFβ-induced transcription. ( a ) C2C12 cells were transfected with three different siRNAs (#1, #2 and #3) targeting mouse OTUB1 (300 pM/10-cm dish each) and lysed 48 h after transfection. Extracts were resolved by SDS-PAGE and immunoblotted with OTUB1 and tubulin antibodies. ( b ) C2C12 cells stably expressing a SMAD3-dependent TGFβ-responsive CAGA-luciferase reporter construct were transfected with iFoxO4 or iOTUB1# 1. Cells were treated with or without 50 pM TGFβ for 6 h before lysis and luciferase activity was measured. Data are represented as mean and error bars indicate s.d. ( n =3). ( c ) HaCaT cells stably expressing shRNA against OTUB1 or transfected with control (−) or OTUB1 siRNA (300 pM/10-cm dish each) for 48 h were lysed, and extracts were resolved by SDS-PAGE and immunoblotted with OTUB1 and GAPDH antibodies. ( d ) HaCaT cells, transfected with human OTUB1 siRNA, human FoxO4 siRNA, or stably expressing OTUB1 shRNA, were treated with 50 pM TGFβ for 4 h before RNA isolation. Relative expression levels of indicated mRNAs were analysed by qRT-PCR. Data are represented as mean and error bars indicate s.d. ( n =6). ( e ) HaCaT cells depleted of human OTUB1 or FoxO4 by RNAi were treated with 50 pM TGFβ for 1 h. TGFβ was then washed off and SB505124 (1 μM) added. RNA was isolated 45 min after TGFβ removal. Relative expression levels of OTUB1 and CTGF mRNAs were analysed by qRT-PCR. Data are represented as mean and error bars indicate s.d. ( n =6). Statistical significance of differences between experimental groups was assessed with Student’s t -test. ** P <0.01 and *** P <0.001. Full size image These results demonstrate that depletion of OTUB1 by two independent RNAi (RNA interference) oligonucleotides in mouse and human cells causes inhibition of TGFβ-induced transcriptional activity. To rule out the possibility that these effects were due to off-target effects of siRNAs , we performed rescue experiments by employing OTUB1 constructs harbouring siRNA -resistant silent mutations. Reintroduction of siRNA -resistant full-length OTUB1 rescued the OTUB1 transcripts to ~70% of the endogenous levels (Fig. 5d). Under these conditions, the inhibition of TGFβ-induced PAI-1 mRNA expression caused by OTUB1 depletion was significantly reversed (Fig. 5d). OTUB1 activity and its impact on SMAD3 ubiquitylation To investigate the molecular mechanisms by which OTUB1 regulates SMAD2/3 function, we generated several OTUB1 mutants. Mutants were selected to either abolish OTUB1 catalytic activity or disrupt the interaction of OTUB1 with phospho-SMAD2/3. The catalytic cysteine of OTUB1, C91, is present in the OTU domain of OTUB1 and forms a catalytic triad with D88 and H265, which come into close contact on protein folding [21] . These three residues were targeted for mutagenesis to potentially disrupt the catalytic activity of OTUB1. The N terminus of OTUB1 harbours a ubiquitin-binding domain, which is deleted in the OTUB1 ΔN mutant [19] , [30] . We also generated several other point mutants of OTUB1 by random mutagenesis; however, only K71R was selected for this study for its suitable properties as discussed below. The relative locations of the key residues mutated for this study are indicated in a schematic representation of OTUB1 ( Fig. 4a , Supplementary Table S1 ). 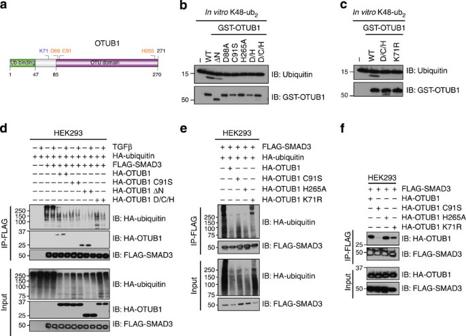Figure 4: Characterization of OTUB1 activityin vitro (a) A schematic representation of OTUB1 indicating the positions of key residues and domains. (b,c) Human recombinant GST-OTUB1 or indicated GST-OTUB1 mutants were incubated with K48-linked di-ubiquitin chains in a DUB assay buffer for 1 h at 30 °C. The reaction was stopped by the addition of 1 × SDS sample buffer and the assay mix was resolved by SDS-PAGE and immunoblotted with GST or ubiquitin antibodies as indicated. (d–f) HEK293 cells were co-transfected with vectors encoding N-terminal HA-tagged OTUB1 or indicated HA-OTUB1 mutants (C91S, ΔN, D88A/C91S/H265A (D/C/H), H265A, K71R) and N-terminal FLAG-tagged SMAD3. Before lysis (in the presence of iodoacetamide), cells were treated with or without 50 pM TGFβ and 10 μM bortezomib for 3 h. FLAG immunoprecipitates (IP) or extracts were resolved by SDS-PAGE and immunoblotted with the indicated antibodies. Figure 4: Characterization of OTUB1 activity in vitro ( a ) A schematic representation of OTUB1 indicating the positions of key residues and domains. ( b , c ) Human recombinant GST-OTUB1 or indicated GST-OTUB1 mutants were incubated with K48-linked di-ubiquitin chains in a DUB assay buffer for 1 h at 30 °C. The reaction was stopped by the addition of 1 × SDS sample buffer and the assay mix was resolved by SDS-PAGE and immunoblotted with GST or ubiquitin antibodies as indicated. ( d – f ) HEK293 cells were co-transfected with vectors encoding N-terminal HA-tagged OTUB1 or indicated HA-OTUB1 mutants (C91S, ΔN, D88A/C91S/H265A (D/C/H), H265A, K71R) and N-terminal FLAG-tagged SMAD3. Before lysis (in the presence of iodoacetamide), cells were treated with or without 50 pM TGFβ and 10 μM bortezomib for 3 h. FLAG immunoprecipitates (IP) or extracts were resolved by SDS-PAGE and immunoblotted with the indicated antibodies. Full size image We assessed the catalytic activity of OTUB1 mutants described above by employing in vitro deubiquitylation assays on di- or polyubiquitin chains. Wild-type OTUB1 cleaved K48-linked diubiquitin ( Fig. 4b ) as well as longer K48-linked polyubiquitin chains ( Supplementary Fig. S3a ), but not K63-linked polyubiquitin chains ( Supplementary Fig. S3b ). OTUB1 ΔN mutant exhibited slightly reduced catalytic activity against K48-linked ubiquitin chains ( Fig. 4b and Supplementary Fig. S3a ), whereas all the other mutants of OTUB1, D88A, C91S, H265A, D88A/H265A (D/H), D88A/C91S/H265A (D/C/H; Fig. 4b ) and K71R ( Fig. 4c ) did not cleave K48-linked diubiquitin chains, indicating that these mutants were catalytically inactive. We also tested their ability to interact with and deubiquitylate SMAD3 in HEK293 cells. To test this, HEK293 cells were transfected with haemagglutinin (HA)-OTUB1 or mutant constructs together with FLAG-SMAD3 and HA ubiquitin. Full-length HA-OTUB1, as well as HA-OTUB1 ΔN interacted with FLAG-SMAD3, whereas HA-OTUB1 C91S and HA-OTUB1 D/C/H mutants did not ( Fig. 4d ). Co-expression of HA-OTUB1 and FLAG-SMAD3 in HEK293 cells resulted in a spontaneous tail phosphorylation of FLAG-SMAD3 even in the absence of TGFβ ( Supplementary Fig. S3c ). This potentially explains the interaction between HA-OTUB1 and FLAG-SMAD3 under overexpression conditions even in the absence of TGFβ ( Fig. 4d and Supplementary Fig. S3c ). HA-OTUB1 H265A and HA-OTUB1 K71R mutants also interacted with FLAG-SMAD3 ( Fig. 4f ). The interaction of HA-OTUB1 and mutants with FLAG-SMAD3 is not influenced in the absence or presence of transfected HA-ubiquitin ( Supplementary Fig. S4a ). When co-expressed with HA-ubiquitin in HEK293 cells, efficient polyubiquitylation was observed in FLAG-SMAD3 IPs independent of TGFβ stimulation ( Fig. 4d,f ). On co-expression with wild-type OTUB1, a significant reduction in polyubiquitylation of FLAG-SMAD3 IPs was observed ( Fig. 4d,e ). However, this reduction was most probably because of the general reduction in polyubiquitin chains observed in extracts when OTUB1, or catalytically inactive mutants of OTUB1 (C91S and H265A), were overexpressed ( Fig. 4d,e ). Overexpression of the OTUB1 K71R mutant, which is also catalytically inactive but still interacts with SMAD3, only caused a moderate decrease in FLAG-SMAD3-polyubiquitylation levels ( Fig. 4e ). Overexpression of OTUB1 also led to a general reduction in global endogenous polyubiquitylation in extracts ( Supplementary Fig. S4a,b ). This loss was not rescued completely by proteasomal inhibitors bortezomib and lactacystin ( Supplementary Fig. S4a,b ). OTUB1 prevents SMAD3 ubiquitylation The general loss of overall polyubiquitylation in whole-cell extracts on OTUB1 overexpression led us to test whether OTUB1 was capable of deubiquitylating polyubiquitylated SMAD2/3. FLAG-SMAD2/3 and SMAD4 overexpressed in HEK293 cells together with HA-ubiquitin and HA-NEDD4L (E3) were immunoprecipitated and used as a substrate for an OTUB1 in vitro deubiquitylation assay. Before lysis, cells were treated with TGFβ and bortezomib to induce SMAD2/3/4 complex formation and inhibit proteasomal degradation, preserving K48-linked polyubiquitin chains, respectively ( Fig. 5a ) [41] . On co-expression in HEK293 cells, NEDD4L induces K48-linked polyubiquitin chains on FLAG-SMAD3 ( Supplementary Fig. S5a ), and E3-mediated degradation of endogenous SMAD2/3 can be rescued by bortezomib ( Supplementary Fig. S5b ). Wild-type OTUB1 and the ΔN mutant, both capable of cleaving K48-linked di- or polyubiquitin chains in vitro , along with all the catalytically inactive mutants (D88A, C91S, H265A, D/H, D/C/H, K71R) were not able to deubiquitylate the polyubiquitylated FLAG-SMAD2/3/4 complex ( Fig. 5a ). Identical results were obtained when in vitro -polyubiquitylated recombinant SMAD3 was used as a substrate for OTUB1 ( Supplementary Fig. S5c ), indicating that OTUB1 does not deubiquitylate polyubiquitylated SMAD3. 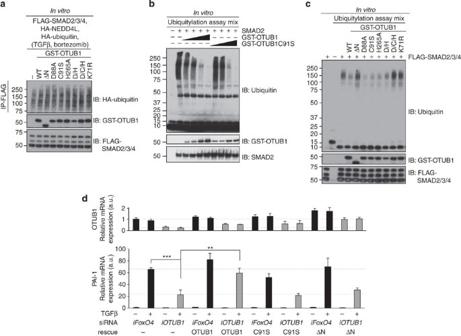Figure 5: OTUB1 prevents SMAD3 ubiquitylationin vitro. (a) For in-cell polyubiquitylation of FLAG-SMAD2/3/4, vectors encoding FLAG-SMAD2/3/4 were co-transfected with HA-NEDD4L and HA-ubiquitin in HEK293 cells and treated with 50 pM TGFβ and 10 μM bortezomib for 3 h before lysis and FLAG-SMAD2/3/4 were immunoprecipitated. Anin vitroDUB assay of in-cell polyubiquitylated FLAG-SMAD2/3/4 was performed with GST-OTUB1 and the indicated GST-OTUB1 mutants in DUB assay buffer for 1 h at 30 °C. The assay mix was resolved by SDS-PAGE and immunoblotted with the indicated antibodies. (b) Anin vitroubiquitylation assay was performed with human recombinant SMAD2. SMAD2 was incubated with E1, E2, E3 and ubiquitin in ubiquitylation assay buffer for 1 h at 30 °C. Increasing concentrations of GST-OTUB1 and GST-OTUB1 C91S (8–60 ng μl−1) were added at the start of the ubiquitylation assay (time 0). Proteins were resolved by SDS-PAGE and immunoblotted with the indicated antibodies. (c) FLAG-SMAD2/3/4 IPs (from HEK293 cells expressing FLAG-SMAD2/3/4 treated with 50 pM TGFβ for 1 h before lysis) were ubiquitylatedin vitroin ubiquitylation assay buffer for 1 h at 30 °C using E1, E2, E3 and ubiquitin. The indicated DUBs were added at the start of the ubiquitylation assay (time 0) and proteins were resolved by SDS-PAGE and immunoblotted with the indicated antibodies. (d) HaCaT cells were stably transfected with vectors encoding siRNA-resistant silent mutations (rescue) of the indicated OTUB1 constructs. These cells were then transfected with control FoxO4 or OTUB1 siRNA for 48 h and treated with or without TGFβ for 4 h before RNA isolation. Relative expression levels of indicated mRNAs were analysed by qRT-PCR. Data are represented as mean and error bars indicate s.d. (n=6). Statistical significance of differences between experimental groups was assessed with Student’st-test. **P<0.01 and ***P<0.001. Figure 5: OTUB1 prevents SMAD3 ubiquitylation in vitro. ( a ) For in-cell polyubiquitylation of FLAG-SMAD2/3/4, vectors encoding FLAG-SMAD2/3/4 were co-transfected with HA-NEDD4L and HA-ubiquitin in HEK293 cells and treated with 50 pM TGFβ and 10 μM bortezomib for 3 h before lysis and FLAG-SMAD2/3/4 were immunoprecipitated. An in vitro DUB assay of in-cell polyubiquitylated FLAG-SMAD2/3/4 was performed with GST-OTUB1 and the indicated GST-OTUB1 mutants in DUB assay buffer for 1 h at 30 °C. The assay mix was resolved by SDS-PAGE and immunoblotted with the indicated antibodies. ( b ) An in vitro ubiquitylation assay was performed with human recombinant SMAD2. SMAD2 was incubated with E1, E2, E3 and ubiquitin in ubiquitylation assay buffer for 1 h at 30 °C. Increasing concentrations of GST-OTUB1 and GST-OTUB1 C91S (8–60 ng μl −1 ) were added at the start of the ubiquitylation assay (time 0). Proteins were resolved by SDS-PAGE and immunoblotted with the indicated antibodies. ( c ) FLAG-SMAD2/3/4 IPs (from HEK293 cells expressing FLAG-SMAD2/3/4 treated with 50 pM TGFβ for 1 h before lysis) were ubiquitylated in vitro in ubiquitylation assay buffer for 1 h at 30 °C using E1, E2, E3 and ubiquitin. The indicated DUBs were added at the start of the ubiquitylation assay (time 0) and proteins were resolved by SDS-PAGE and immunoblotted with the indicated antibodies. ( d ) HaCaT cells were stably transfected with vectors encoding siRNA-resistant silent mutations (rescue) of the indicated OTUB1 constructs. These cells were then transfected with control FoxO4 or OTUB1 siRNA for 48 h and treated with or without TGFβ for 4 h before RNA isolation. Relative expression levels of indicated mRNAs were analysed by qRT-PCR. Data are represented as mean and error bars indicate s.d. ( n =6). Statistical significance of differences between experimental groups was assessed with Student’s t -test. ** P <0.01 and *** P <0.001. Full size image This led us to hypothesize that OTUB1 might inhibit the ubiquitylation of SMAD2/3. The ability of OTUB1 to inhibit the ubiquitylation of target proteins independent of its catalytic activity has been reported before [30] . We polyubiquitylated recombinant SMAD2 in vitro using UBE1 (E1), UBE2D1 (E2) and NEDD4L (E3) (refs 14 , 42 ) ( Fig. 5b ). OTUB1 or OTUB1 C91S were added at increasing doses at the start of the reaction. In the absence of SMAD2, no autoubiquitylation of E2 or E3 is detected ( Fig. 5b ; lane 1). In the presence of SMAD2, robust polyubiquitylation is observed ( Fig. 5b ; lane 2). Adding increasing amounts of wild-type OTUB1 or catalytically inactive OTUB1 C91S at the start of the assay inhibits polyubiquitylation of SMAD2 in a dose-dependent manner ( Fig. 5b ; lanes 3–10). We also tested the ability of OTUB1 and mutants to inhibit the polyubiquitylation of FLAG-SMAD2/3/4 in vitro . As seen with recombinant SMAD2, TGFβ-treated FLAG-SMAD2/3/4 IPs were polyubiquitylated in the presence of E1, E2 and E3. Polyubiquitylation was significantly inhibited when OTUB1 and most of the OTUB1 mutants (D88A, C91S, H265A, D/H) were added at the start of the ubiquitylation assay ( Fig. 5c ; lanes 4, 6–9). However, OTUB1 ΔN, D/C/H and K71R were unable to inhibit polyubiquitylation ( Fig. 5c ; lanes 5, 10 and 11). These results imply that OTUB1 inhibits the ubiquitylation of SMAD2/3 rather than directly deubiquitylating them. Consequently, we investigated how OTUB1 has an impact on the TGFβ-induced transcription. We tested whether the catalytic activity of OTUB1, its ability to inhibit ubiquitylation of SMAD2/3 or its ability to interact with SMAD3 are essential to enhance TGFβ-induced transcription. As described previously, the loss in expression of the TGFβ target gene PAI-1 caused by siRNA -mediated depletion of OTUB1 is rescued by reintroduction of siRNA -resistant OTUB1 ( Fig. 5d , Supplementary Fig. S5d ). However, neither OTUB1 C91S (catalytically inactive, inhibits polyubiquitylation of SMAD3 in vitro but does not interact with SMAD3) nor OTUB1 ΔN (catalytically active and interacts with SMAD3 but does not inhibit polyubiquitylation of SMAD3 in vitro ) were able to rescue PAI-1 expression ( Fig. 5d ). This suggests that the ability of OTUB1 to both interact with and prevent the ubiquitylation of SMAD3 independent of its catalytic activity are essential for the regulation of TGFβ-induced transcription. OTUB1 prevents transfer of ubiquitin from E2s to E3s OTUB1 has previously been reported to inhibit ubiquitylation of target proteins by interacting with and inhibiting E2 ubiquitin-conjugating enzymes [29] , [30] , [31] , [32] . Consistent with the reported findings [30] , we were able to identify E2 ubiquitin-conjugating enzymes, including UBE2N and all members of UBE2D and UBE2E family of E2s, as major interactors of GFP-OTUB1 by mass spectrometry ( Supplementary Fig. S6 and Supplementary Table S2 ). In addition, we identified UBE2V1/2 and UBE2L3 as novel interactors of OTUB1 ( Supplementary Table S2 ). Further, in endogenous OTUB1 IPs we were able to detect endogenous UBE2D and UBE2N independent of TGFβ signalling ( Fig. 6a ). To investigate whether the inhibition of E2 by OTUB1 was the rate-limiting step in its inhibition of SMAD3 polyubiquitylation in vitro , we set up an in vitro ubiquitylation assay with ubiquitin, E1, varying concentrations of E2, E3 and recombinant human SMAD3 in the presence or absence of 0.5 μM GST-OTUB1 ( Fig. 6b ). In the absence of OTUB1, increasing concentrations of E2 resulted in enhanced polyubiquitylation of SMAD3 in a dose-dependent manner ( Fig. 6b ). As observed previously ( Fig. 5b,c ), the presence of OTUB1 in the reaction resulted in a significant inhibition of polyubiquitylation especially at lower concentrations of E2 ( Fig. 6b ). Higher concentrations of E2 substantially rescued this inhibition suggesting that binding of OTUB1 to E2 is likely to be the rate-limiting step in the inhibition of polyubiquitylation of SMAD3 ( Fig. 6b ). We next investigated whether OTUB1 inhibits E2 by preventing the conjugation of ubiquitin or the transfer of ubiquitin from E2 to E3. In the presence of ubiquitin, ATP and E1, almost every molecule of E2 becomes loaded with ubiquitin ( Fig. 6c ; compare lane 1 with 2). This ubiquitin loading of E2 is not inhibited when wild-type OTUB1, OTUB1 C91S or OTUB1 K71R mutants are present. When E3 ligase NEDD4L and its substrate SMAD3 are added to the reaction, in the absence of OTUB1 most of the ubiquitin at the predicted molecular weight disappears ( Fig. 6c ; compare lane 2 with 7). Under these conditions, consistent with an efficient transfer of ubiquitin from E2-Ub to E3 and substrate, the E2 is mostly observed in a non-ubiquitin-loaded native molecular weight state ( Fig. 6c ). However, when wild-type OTUB1 is added to the reaction at the start, some ubiquitin is observed at its native molecular weight, whereas a significant amount of ubiquitin-loaded E2 is also observed, suggesting that OTUB1 inhibits the transfer of ubiquitin from the E2-Ub complex to E3 ( Fig. 6c ). 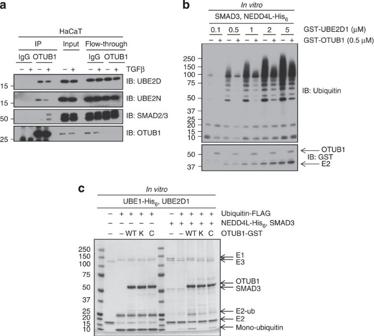Figure 6: OTUB1 interacts with E2 enzymes and inhibits efficient ubiquitin transfer from E2 to E3. (a) An endogenous IP with OTUB1 antibody or pre-immune sheep IgG was performed in HaCaT cell extracts stimulated with or without 50 pM TGFβ for 1 h before lysis in the presence of dithiobis[succinimidyl propionate] (DSP). Cell extracts (input), endogenous IgG or OTUB1 IPs and the corresponding immune-depleted flow-through extracts were resolved by SDS-PAGE and immunoblotted with the indicated antibodies. (b) Anin vitroubiquitylation assay was performed with human recombinant SMAD3, His-E1 (0.1 μM), ubiquitin, His-E3 (1 μM) and increasing concentrations of GST-E2 (0.1–5 μM) in ubiquitylation assay buffer for 1 h at 30 °C. GST-OTUB1 was added at the start of the ubiquitylation assay (time 0). Proteins were resolved by SDS-PAGE and immunoblotted with the indicated antibodies. (c) His-E1, E2, FLAG-ubiquitin, GST-OTUB1 and mutants were mixed with or without His-E3 and SMAD3 before the addition of ATP. After 10 min at 30 °C, proteins were separated by SDS-PAGE and visualized with Coomassie Instantblue. Figure 6: OTUB1 interacts with E2 enzymes and inhibits efficient ubiquitin transfer from E2 to E3. ( a ) An endogenous IP with OTUB1 antibody or pre-immune sheep IgG was performed in HaCaT cell extracts stimulated with or without 50 pM TGFβ for 1 h before lysis in the presence of dithiobis[succinimidyl propionate] (DSP). Cell extracts (input), endogenous IgG or OTUB1 IPs and the corresponding immune-depleted flow-through extracts were resolved by SDS-PAGE and immunoblotted with the indicated antibodies. ( b ) An in vitro ubiquitylation assay was performed with human recombinant SMAD3, His-E1 (0.1 μM), ubiquitin, His-E3 (1 μM) and increasing concentrations of GST-E2 (0.1–5 μM) in ubiquitylation assay buffer for 1 h at 30 °C. GST-OTUB1 was added at the start of the ubiquitylation assay (time 0). Proteins were resolved by SDS-PAGE and immunoblotted with the indicated antibodies. ( c ) His-E1, E2, FLAG-ubiquitin, GST-OTUB1 and mutants were mixed with or without His-E3 and SMAD3 before the addition of ATP. After 10 min at 30 °C, proteins were separated by SDS-PAGE and visualized with Coomassie Instantblue. Full size image OTUB1 C91S, a catalytically inactive mutant that does not interact with SMAD3 but prevents its ubiquitylation, mimics wild-type OTUB1. However, OTUB1 K71R, a catalytically inactive mutant, does not appear to inhibit the transfer of ubiquitin from the E2-Ub complex to E3 ( Fig. 6c cf. bottom line mono-ubiquitin). This is consistent with the inability of OTUB1 K71R mutant to inhibit the ubiquitylation of SMAD3 ( Fig. 5c ). These results suggest that by binding to E2 ubiquitin-conjugating enzymes, OTUB1 appears to inhibit the transfer of ubiquitin from E2-Ub complex onto E3 ubiquitin ligases. OTUB1 rescues phospho-SMAD2/3 from proteasomal degradation We have demonstrated that OTUB1 binds to phospho-SMAD2/3 and E2 ubiquitin-conjugating enzymes, thereby inhibiting the polyubiquitylation of SMAD2/3 in vitro. Therefore, we reasoned that OTUB1 enhances the TGFβ-induced transcriptional responses by stabilization of the active phospho-SMAD2/3 pool in cells by protecting it from polyubiquitin-mediated proteasomal degradation. To demonstrate that the turnover of active phospho-SMAD2/3 is mediated in part by proteasomal degradation, HaCaT cells were treated with 26S proteasome inhibitors (bortezomib or MG132) and TGFβ for 3 h. Bortezomib, and to a lesser extent MG132, treatment resulted in enhanced levels of TGFβ-induced phospho-SMAD2/3 as well as polyubiquitylated proteins ( Supplementary Fig. S7a ). However, when TGFβ and bortezomib were added to the cells for 1 h, the increase in the levels of TGFβ-induced phospho-SMAD2/3 caused by bortezomib was only slight. In addition, early induction of phospho-SMAD2/3 by TGFβ was unaffected by siRNA-mediated depletion of OTUB1 ( Fig. 7a ). As polyubiquitylation and degradation of phospho-SMAD2/3 occurs subsequent to the assembly of the active SMAD2/3/4 complex at the transcription sites [14] , we performed a pulse-chase experiment. Control or OTUB1-depleted HaCaT cells were stimulated with TGFβ for 1 h to induce maximal phosphorylation of SMAD2/3, after which the TGFβ ligand was removed. The levels of phospho-SMAD2/3 were tracked at fixed time points thereafter in the presence or absence of bortezomib. The cells depleted of OTUB1 expression exhibited lower levels of phospho-SMAD2/3 after 30 min and 1 h of TGFβ removal compared with control cells ( Fig. 7b ; lanes 2 and 6). This effect appeared to be a result of rapid proteasomal degradation, as the levels of phospho-SMAD2/3 are stabilized in the presence of the proteasomal inhibitor bortezomib ( Fig. 7b ; lanes 4 and 8). The levels of total SMAD2/3 or SMAD4 did not change significantly ( Fig. 7b ). Bortezomib stabilized phospho-SMAD2/3 levels for up to 16 h following ligand removal ( Supplementary Fig. S7b ). The reduction in the levels of phospho-SMAD2 caused by depletion of OTUB1 was rescued by a siRNA -resistant wild-type FLAG-OTUB1 construct, suggesting that the results obtained were unlikely to be due to the off-target effects ( Fig. 7c ). 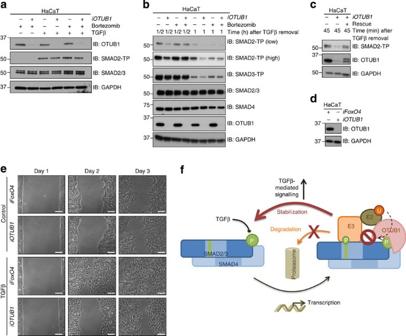Figure 7: OTUB1 protects phospho-SMAD2/3 from proteasomal degradation and has an impact on TGFβ-induced cell migration. (a) HaCaT cells transfected withFoxO4(−) orOTUB1siRNAs were treated with TGFβ (50 pM) and bortezomib (10 μM) for 1 h. Extracts were resolved by SDS-PAGE and immunoblotted with the indicated antibodies. (b) HaCaT cells, expressing control shRNA (−) or OTUB1 shRNA were transfected withFoxO4(−) orOTUB1siRNAs, respectively, 48 h before cell lysis. Cells were serum starved for 16 h and stimulated with TGFβ (50 pM) and bortezomib (10 μM) for 1 h. The cells were then washed in PBS and media was replaced with starvation media supplemented with SB505124 (1 μM; to block any further TGFβ receptor activity), with or without bortezomib (10 μM). The cells were lysed at ½ or 1 h time points and cell extracts resolved by SDS-PAGE and immunoblotted with the indicated antibodies. (c) As inb, except cells were transfected with vector encoding FLAG-tagged full-length OTUB1 resistant to OTUB1 shRNAs and siRNAs (rescue). (d) HaCaT cells used inewere lysed after 48 h and extracts were resolved by SDS-PAGE and immunoblotted with the indicated antibodies, confirming a knockdown of OTUB1. (e) HaCaT cells stably expressing control shRNA andFoxO4siRNA or OTUB1 shRNA andOTUB1siRNA were seeded onto migration inserts (Ibidi). After 24 h, the inserts were removed and cells were serum starved for 4 h and stimulated without or with TGFβ (50 pM). Cell migration was tracked by taking images of the gaps every 24 h. Scale bars, 100 μm. (f) A schematic representation of OTUB1 function within the TGFβ signalling pathway. TGFβ induces SMAD2/3 tail phosphorylation, association with SMAD4 and entry into the nucleus, where SMADs act as transcription factors. Following linker phosphorylation, E3 ubiquitin ligase NEDD4L recognizes the SMAD2/3/4 complex and polyubiquitylates SMAD2/3, leading to proteasomal degradation. OTUB1 interacts with, and thereby chaperones, the active SMAD2/3 complex by inhibiting its ubiquitylation, through its interactions with and inhibition of cognate E2. Proteasomal degradation of active SMAD2/3 is thus prevented and the complex can recycle, which leads to sustained TGFβ signalling. Figure 7: OTUB1 protects phospho-SMAD2/3 from proteasomal degradation and has an impact on TGFβ-induced cell migration. ( a ) HaCaT cells transfected with FoxO4 (−) or OTUB1 siRNAs were treated with TGFβ (50 pM) and bortezomib (10 μM) for 1 h. Extracts were resolved by SDS-PAGE and immunoblotted with the indicated antibodies. ( b ) HaCaT cells, expressing control shRNA (−) or OTUB1 shRNA were transfected with FoxO4 (−) or OTUB1 siRNAs, respectively, 48 h before cell lysis. Cells were serum starved for 16 h and stimulated with TGFβ (50 pM) and bortezomib (10 μM) for 1 h. The cells were then washed in PBS and media was replaced with starvation media supplemented with SB505124 (1 μM; to block any further TGFβ receptor activity), with or without bortezomib (10 μM). The cells were lysed at ½ or 1 h time points and cell extracts resolved by SDS-PAGE and immunoblotted with the indicated antibodies. ( c ) As in b , except cells were transfected with vector encoding FLAG-tagged full-length OTUB1 resistant to OTUB1 shRNAs and siRNAs (rescue). ( d ) HaCaT cells used in e were lysed after 48 h and extracts were resolved by SDS-PAGE and immunoblotted with the indicated antibodies, confirming a knockdown of OTUB1. ( e ) HaCaT cells stably expressing control shRNA and FoxO4 siRNA or OTUB1 shRNA and OTUB1 siRNA were seeded onto migration inserts (Ibidi). After 24 h, the inserts were removed and cells were serum starved for 4 h and stimulated without or with TGFβ (50 pM). Cell migration was tracked by taking images of the gaps every 24 h. Scale bars, 100 μm. ( f ) A schematic representation of OTUB1 function within the TGFβ signalling pathway. TGFβ induces SMAD2/3 tail phosphorylation, association with SMAD4 and entry into the nucleus, where SMADs act as transcription factors. Following linker phosphorylation, E3 ubiquitin ligase NEDD4L recognizes the SMAD2/3/4 complex and polyubiquitylates SMAD2/3, leading to proteasomal degradation. OTUB1 interacts with, and thereby chaperones, the active SMAD2/3 complex by inhibiting its ubiquitylation, through its interactions with and inhibition of cognate E2. Proteasomal degradation of active SMAD2/3 is thus prevented and the complex can recycle, which leads to sustained TGFβ signalling. Full size image TGFβ signalling has a critical role in multiple cellular processes, including wound healing and migration [3] , [43] , [44] , [45] . The induction of cellular migration by TGFβ is in part implicated in cancer progression and metastasis [3] , [45] . To assess the impact of OTUB1 on TGFβ-induced cellular migration, a wound-healing ‘scratch assay’ was employed. Control or OTUB1-depleted HaCaT cells ( Fig. 7d ) were cultured to confluency in adjacent chambers of an insert separated by a small fixed-sized spacer. On removal of the insert, a uniform gap was formed. Cellular migration onto the gap was monitored for up to 48 h ( Fig. 7e ). In control cells, TGFβ treatment induced migration of cells within 24 h, and by 48 h the gap was completely covered with cells. Depletion of OTUB1 substantially inhibited the migration of HaCaT cells onto the gap after TGFβ treatment ( Fig. 7e ). This study uncovers an intriguing regulatory role for OTUB1 in recognizing TGFβ-induced phospho-SMAD2/3, controlling their turnover and consequently modulating pathway signalling. The results reveal for the first time a remarkable interplay between phosphorylation and the recruitment of OTUB1 to its target in the TGFβ pathway. The findings shed light into the molecular mechanisms by which the phospho-SMAD2/3–OTUB1 interaction results in the regulation of TGFβ-induced transcription as well as phospho-SMAD2/3 turnover. TGFβ-induced phosphorylation of SMAD2/3 by the type I TGFβ receptor kinases is a fundamental feature in the intracellular transduction of TGFβ ligands. This induces the formation of an active SMAD2/3/4 transcription complex, translocation to the nucleus and transcriptional control of target genes [5] . OTUB1 was isolated from a proteomic screen as an interactor of GFP-SMAD3 only when cells were treated with TGFβ. Remarkably, endogenous OTUB1 interacts with SMAD2/3 only on TGFβ induction ( Fig. 1b,d ), and the levels of phospho-SMAD2/3 on TGFβ stimulation directly correlate with the ability of OTUB1 to pull down SMAD2/3 ( Fig. 1c ). SMAD4 was also detected in OTUB1 immunoprecipitates on TGFβ stimulation ( Fig. 1b ). However, even in the absence of SMAD4, OTUB1 interacts with TGFβ-induced phospho-SMAD2/3, indicating that SMAD4 is not necessary to mediate phospho-SMAD2/3–OTUB1 interaction ( Fig. 2a ). Consistent with the notion that OTUB1 interaction could be phospho-SMAD2/3-dependent, dephosphorylation of OTUB1 IPs by λ-phosphatase to dephosphorylate phospho-SMAD2/3 partially abolishes OTUB1–SMAD2/3 interaction ( Fig. 2b ). Further, a SMAD2 tail phospho-peptide was able to interact with recombinant OTUB1 as well as endogenous OTUB1 from extracts indicating that tail phosphorylation of SMAD2 is sufficient for its interaction with OTUB1 ( Fig. 2c,d ). Despite the phospho-dependent nature of OTUB1 interaction with SMAD2/3, no phospho-interaction motifs within OTUB1 have been reported. A phospho-SMAD3–OTUB1 structural analysis might shed light into the molecular basis of their interaction. To date, no phospho-dependent mode of OTUB1 recruitment to its target has been reported. The TGFβ-dependent recruitment of OTUB1, a DUB, combined with the inhibition of TGFβ-induced transcriptional responses on OTUB1 depletion initially suggested that OTUB1 might have an impact on TGFβ signalling by deubiquitylating and stabilizing phosho-SMAD2/3 in cells. It is known that SMAD2/3-TP in the nucleus are targeted for polyubiquitylation by NEDD4L on further phosphorylation at the linker region by CDK8/9, which then leads to their proteasomal degradation ( Supplementary Fig. S5a,b ) [14] . In vitro OTUB1 cleaves K48-linked polyubiquitin chains, which in cells direct target proteins for proteasomal degradation [46] . However, OTUB1 was unable to deubiquitylate polyubiquitylated SMAD2/3 in vitro ( Fig. 5a ). Further investigations revealed that the action of OTUB1 predominantly relies on its ability to inhibit the ubiquitylation of SMAD2/3 in vitro rather than isopeptide cleavage ( Fig. 5b,c ). Further, some catalytically inactive mutants of OTUB1, including OTUB1 C91S, were also able to inhibit SMAD2/3 ubiquitylation in vitro ( Fig. 5c ). The ability of OTUB1 to inhibit the polyubiquitylation of chromatin on DNA damage independent of its catalytic activity has been shown previously [30] . This and other studies have reported that OTUB1 inhibits ubiquitylation by binding to and inhibiting E2 enzymes [25] , [29] , [30] , [31] , [32] . In agreement with these reports, we identified several E2 enzymes, including UBE2D1, as OTUB1-interacting partners from a proteomic screen. Moreover, we demonstrated the endogenous interactions between OTUB1 and UBE2N or UBE2D1 ( Fig. 6a ). We further showed that OTUB1, by binding to UBE2D1, inhibits the transfer of ubiquitin from E2-Ub conjugate to E3 ubiquitin ligase NEDD4L and subsequently to SMAD3 ( Fig. 6c ). The activation of TGFβ signalling results in the transcription of target genes, which ultimately determines the nature of cellular responses. Our findings indicate that OTUB1 modulates TGFβ-induced transcriptional responses. RNAi -mediated depletion of OTUB1 from HaCaT cells resulted in inhibition of TGFβ-induced expression of PAI-1 and CTGF transcripts, both known TGFβ target genes ( Fig. 3d,e ) [47] , [48] . We were able to rescue the inhibition of TGFβ-induced transcription on OTUB1 depletion by siRNA -resistant OTUB1 ( Fig. 5d ). However, neither siRNA -resistant OTUB1 C91S mutant (catalytically inactive, SMAD3-interaction deficient but able to inhibit SMAD3 ubiquitylation) nor OTUB1 ΔN mutant (catalytically active, interacts with SMAD3 but unable inhibit SMAD3 ubiquitylation) was able to rescue TGFβ-induced transcription caused by OTUB1 depletion ( Fig. 5d ). Together, these results imply that binding to SMAD2/3 as well as the ability to inhibit SMAD2/3 ubiquitylation are essential for OTUB1 to have an impact on the TGFβ pathway. Therefore, the association of OTUB1 with phospho-SMAD2/3 would be predicted to prevent SMAD2/3 from being polyubiquitylated and degraded, thereby enhancing TGFβ signalling. Consistent with this notion, the depletion of OTUB1 from cells leads to a rapid loss in levels of SMAD2/3-TP but the loss in levels are rescued on treatment of cells with proteasomal inhibitor bortezomib or expression of siRNA -resistant OTUB1 ( Fig. 7b,c ). In this study, we have identified OTUB1 as a novel regulator of the TGFβ pathway. The TGFβ pathway controls multiple cellular processes and is implicated in carcinogenesis, in part through the induction of cellular migration [3] , [45] . We demonstrate that the depletion of OTUB1 from HaCaT cells significantly inhibits lateral migration induced by TGFβ ( Fig. 7e ). Our findings imply that OTUB1 enhances TGFβ signalling responses by interacting with and stabilizing SMAD2/3-TP, by preventing its ubiquitylation and degradation ( Fig. 7f ). These observations make OTUB1 a promising target for the development of small molecule inhibitors specifically targeting the OTUB1–SMAD2/3 interaction against diseases, such as cancer and fibrosis, where TGFβ signalling is abnormal. Cell culture All cells (HaCaT, HEK293, SW480, U2OS, C2C12) were cultured in DMEM (Gibco) supplemented with 10% fetal bovine serum (Hyclone), 2 mM L -Glutamine (Lonza) and 1% penicillin/streptomycin (Lonza) and maintained at 37 o C in a humidified atmosphere with 5% CO 2 . HEK293 cells were obtained from ATCC, HaCaT cells from J. Massague (New York), U2OS cells from J. Rouse (Dundee), SW480 cells from A. Prescott (Dundee) and C2C12 cells from G. Inman (Dundee). Primary cells (MEFs and BMDMs) were generated from animals that were housed under specific pathogen-free conditions in accordance with UK and EU regulations. Wild-type MEFs were isolated from decapitated embryos with red organs removed. The embryo was minced and resuspended in 1 ml trypsin and incubated at 37 °C for 15 min before the addition of 10 ml growth medium. Cells were plated and allowed to attach overnight before cells were washed with fresh medium to remove debris. Growth media were additionally supplemented with Na-pyruvate and non-essential amino acids. BMDMs were generated by flushing femurs from a female mouse with PBS. Cells were then pelleted by centrifugation and cultured on bacterial grade plastic plates for 7 days in media (additionally supplemented 0.25 μg ml −1 amphotericin and 5 ng ml −1 recombinant macrophage colony-stimulating factor (M-CSF)). Cells were then detached by scraping in versene (Invitrogen) and re‐plated on tissue culture-treated petri dishes. All procedures were carried out in accordance with University of Dundee and United Kingdom Home Office regulations [49] , [50] . FlpIN TRex HEK293 cell lines (Invitrogen) stably expressing tetracycline inducible GFP constructs (GFP, GFP-SMAD1, GFP-SMAD3 and GFP-OTUB1) were additionally grown in 100 μg ml −1 hygromycin B and 15 μg ml −1 blasticidin. GFP-protein expression was induced with 20 ng ml −1 doxycycline for 16 h before lysis. Stable cell lines infected with pBABE-puro (Cell Biolabs Inc.) retroviral constructs or pSUPERIOR-puro retroviral (Oligoengine) shRNA constructs were supplemented with 2 μg ml −1 puromycin. Stable CAGA (TGFβ responsive) luciferase reporter C2C12 cells (obtained from Dr G. Inman) were selected in 0.7 mg ml −1 G418 (Sigma). Cells were serum starved for 16 h at 37 o C before ligand treatment with human recombinant BMP 2 (25 ng ml −1 ) or TGFβ 1 (50 pM; R&D Systems) for the indicated time points. SB505124 (Sigma), a specific TGFβ-receptor ALK4/5/7 inhibitor, was used at 1 μM for the indicated time points [51] . Proteasome inhibitors bortezomib (LC Laboratories), MG132 (Calbiochem) and lactacystin (Sigma) were used at 10 μM for 3 h. Plasmid transfections were done using 25 μl of 1 mg ml −1 polyethylenimine (Polysciences, in 25 mM HEPES pH 7.5) in 1 ml DMEM with a maximum of 10 μg plasmid DNA [52] . All plasmids expressing mammalian proteins were cloned into pCMV5, pBABE-puro or pCDNA-Frt-TO vectors with N-terminal FLAG, GFP or HA tags. pCDNA-Frt-TO plasmids were used to generate stable tetracycline inducible HEK293 cell lines following the manufacturer’s protocol (Invitrogen). pRetro SUPERIOR shRNA control or OTUB1 shRNA (5′-GCAAGTTCTTCGAGCACTT-3′), as well as pBABE constructs (pBABE-puro control or OTUB1 or mutant constructs harbouring silent mutations for protection against human iOTUB1#1 and/or #3 siRNAs ) were generated as retroviruses in HEK293T cells according to manufacturers’ protocols and used to infect target cells [53] . Infected cells were selected and maintained in 2 μg ml −1 puromycin. All DNA constructs used were verified by DNA sequencing, performed by DNA Sequencing & Services (MRCPPU, College of Life Sciences, University of Dundee, Scotland, http://www.dnaseq.co.uk ) using Applied Biosystems Big-Dye Ver 3.1 chemistry on an Applied Biosystems model 3730 automated capillary DNA sequencer. For siRNA oligonucleotide transfections, the cells were transfected during attachment. Thirty microlitres of transfectin (Bio-Rad) and 300 pM of siRNA (per 10-cm diameter dish) were mixed in 2 ml OptiMEM (Life Technologies). After incubating for 15 min, the solution was added to the cells and cells were lysed 48 h after transfection. The following siRNA oligonucleotides (Sigma) were used: OTUB1 (#1) : human: 5′-GCAAGUUCUUCGAGCACUU-3′, mouse: 5′-GAACCCAUGUGCAAGGAGA-3′, OTUB1 (#3): human: 5′-CCGACUACCUUGUGGUCUA-3′, mouse: 5′-CAAUUGAAGACUUCCACAA-3′, FoxO4: human: 5′-CCCGACCAGAGAUCGCUAA-3′, mouse: 5′-GCAAGUUCAUCAAGGUUCA-3′. FoxO4 siRNA was used as a control as it is known not to interfere with the BMP/TGFβ pathway [33] , [54] . For lysis, cells were scraped on ice in lysis buffer (50 mM Tris–HCl pH 7.5, 0.27 M sucrose, 150 mM NaCl, 1 mM EGTA, 1 mM EDTA, 1 mM sodium orthovanadate, 1 mM sodium β-glycerophosphate, 50 mM sodium fluoride, 5 mM sodium pyrophosphate, 1% Triton X-100 and 0.5% Nonidet P-40) supplemented with complete protease inhibitors (one tablet per 25 ml; Roche) and 0.1% β-mercaptoethanol (Sigma) or 50 mM iodoacetamide (Sigma) or 2.5 mg ml −1 dithiobis[succinimidyl propionate] (DSP) (Thermo Scientific). Lysates were cleared and processed immediately or snap frozen in liquid nitrogen and stored at −80 °C. The protein concentration was determined with a photo spectrometer using Bradford protein assay reagent (Pierce). For RNA isolation, cells were processed using an RNA extraction kit according to the manufacturer’s instructions (Qiagen RNeasy kit). To assay luciferase reporter activity, cells were lysed in passive lysis buffer (Promega), and luciferase activity was measured on a MicroLumat plus LB 96V luminometer from Berthold Technologies. The luciferase counts were normalized to the protein concentration and averaged. Mouse tissue isolation Tissues from mice were frozen in liquid nitrogen and grounded with mortar and pestle. Powdered tissues were resuspended in tissue lysis buffer (10 mM Tris–HCl pH 8, 150 mM NaCl, 1 mM EDTA, 1% NP40, 0.1% SDS and protease inhibitors) and incubated on ice for 30 min before centrifugation. The cleared extracts were processed as described for cell extracts. Immunoprecipitation (IP) Cleared cell extracts were mixed with FLAG-agarose beads, HA-agarose beads, GFP-Trap agarose beads (Chromatek) or antibody-coupled protein G-sepharose beads for 2 h at 4 °C on a rotating platform. The flow-through was retained for western blot analysis and the beads were washed twice in lysis buffer containing 0.4 M NaCl, and twice in buffer A (50 mM Tris–HCl pH 7.5, 0.1 mM EGTA). IP samples, as well as flow-through and input samples, were reduced in SDS sample buffer (62.5 mM Tris–HCl pH 6.8, 10% (v/v) glycerol, 2% (w/v) SDS, 0.02% (w/v) bromophenol blue, 5% (v/v) β-mercaptoethanol) and heated at 95 °C for 5 min. Where appropriate, λ-phosphatase (1 μM) was added to OTUB1 IPs resuspended in 50 μl buffer (50 mM HEPES, 100 mM NaCl, 0.01% Brij-35, 2 mM dithiothreitol (DTT), 1 mM MnCl 2 , pH 7.5) or whole-cell extracts and mixed at 30 °C for 30 min. IPs were then washed and processed as stated above. SDS-PAGE and western blotting Reduced protein extracts (20 μg protein unless stated otherwise) or IPs were separated on 10% SDS-PAGE gels, 4–20% TGX gels (Bio-Rad) or 4–12% NuPAGE bis-tris gels (Invitrogen) by electrophoresis and transferred to polyvinylidene fluoride membranes (Millipore). Membranes were blocked in 5% (w/v) non-fat milk in TBS-T (50 mM Tris–HCl pH 7.5, 150 mM NaCl, 0.2% Tween-20), incubated overnight at 4 °C in 5% milk-TBS-T or 3% BSA-TBS-T with the appropriate primary antibodies followed by incubation with horseradish peroxidase (HRP)-conjugated secondary antibodies in 5% milk-TBS-T and detection by ECL luminescence (Thermo Scientific). Full scans of key western blots are provided in Supplementary Fig. S8 . Antibodies Anti-phospho-Ser463/465 SMAD1 (SMAD1-TP; number 9511), anti-phospho-Ser465/467 SMAD2 (SMAD2-TP; number 3101), anti-SMAD2/3 (number 3102), anti-SMAD4 (number 9515) and anti-GAPDH (number 2118) antibodies were obtained from Cell Signalling. Anti-phospho-Ser423/425 SMAD3 (SMAD3-TP; number 600-401-919) and anti-phospho-Thr179 SMAD3 (SMAD3-LP; number 600-401-C48S) were purchased from Rockland. Anti-SMAD7 (number MAB2029) was from R&D Systems, anti-tubulin from Calbiochem (number DM1A) and anti-ubiquitin from Dako (number Z0458). Anti-K48 ubiquitin (clone Apu2; number 05-1307) was from Millipore. Human recombinant SMAD1(141-268) polypeptide and full-length OTUB1 were used as immunogens in sheep to generate anti-SMAD1 and anti-OTUB1 antibodies, respectively. HRP-conjugated FLAG-(number A8592), HA-(number 12013819001) and GST-(number ab3416) antibodies were from Sigma, Roche and Abcam, respectively. For western blot analysis, all primary antibodies were used at 1:1,000 dilution, except for FLAG, GST, tubulin and GAPDH antibodies, which were used at 1:5,000 dilution. HRP-coupled secondary antibodies (1:5,000) were obtained from Pierce and HRP-coupled light chain-specific secondary antibodies (1:10,000) were purchased from Jackson Immuno Research. Peptide binding assay Biotin-C6-RQTVTSTPCWIELHLNGPLQWLDKVLTQMGSPSVRCS-Sp-M-Sp (SMAD2-TP; 3 μg) was incubated with purified GST-OTUB1 (5 μg) or pre-cleared HaCaT cell lysate (150 μg; with or without pre-treatment with TGFβ (50 pM, 1 h)) in lysis buffer for 30 min, 30 °C, 900 r.p.m. As a control, the phospho-peptide was additionally treated with λ-phosphatase (18 μM) in buffer (50 mM HEPES, 100 mM NaCl, 0.01% Brij-35, 2 mM DTT, 1 mM MnCl 2 pH 7.5). Streptavidin-Sepharose High Performance beads (GE Healthcare) were equilibrated in lysis buffer and 20 μl of 50/50 slurry beads were added for 15 min, 30 °C, 1,300 r.p.m. IPs were washed six times in lysis buffer with 0.4 M NaCl and twice in buffer A. Proteins were resolved by SDS-PAGE and immunoblotted (IB). Mass spectrometry For mass spectrometric analysis, HEK293 cells expressing the protein of interest were lysed in HEPES lysis buffer (40 mM HEPES pH 7.4, 120 mM NaCl, 1 mM EDTA, 10 mM sodium pyrophosphate, 50 mM sodium fluoride, 1.5 mM sodium orthovanadate, 1% Triton X-100) supplemented with 0.5 μM microcystin-LR, 2.5 mg ml −1 dithiobis[succinimidyl propionate] (DSP) and complete protease inhibitors (one tablet per 25 ml). The lysate was incubated for 30 min on ice and the crosslinking reaction was quenched by the addition of Tris–HCl pH 7.4 (200 mM final). Lysates were then cleared by centrifugation (15,000 r.p.m., 30 min) and filtration (0.45 μm). Subsequently, the lysates were incubated with Protein A-agarose beads (1 h on a rotating platform at 4 °C) to limit unspecific binding. The cleared lysate (50 mg) was incubated with GFP-Trap beads (50 μl) for 4 h on a rotating platform at 4 °C. The beads were washed four times in complete lysis buffer containing 0.4 M NaCl and twice in 10 mM Tris–HCl, pH 7.4. The beads were reconstituted in 1 × LDS (Invitrogen) containing 0.1 M DTT, incubated at 37 °C for 1 h and heated at 95 °C for 5 min. The samples were separated by gel electrophoresis, stained with Colloidal Coomassie (Invitrogen) and prepared for mass fingerprinting. Peptide mass fingerprinting data analysis was performed using OLMAT ( http://www.proteinguru.com/MassSpec/OLMAT ). Real-time qRT-PCR HaCaT cells were seeded in six-well plates, transfected with siRNAs and serum starved for 16 h before TGFβ (50 pM) treatment. Complementary DNA was made from 1 μg of the isolated RNA using the I-Script cDNA kit (Bio-Rad) according to the manufacturer’s protocol. qRT-PCR reactions were performed in quadruplicates according to the manufacturer’s protocol in a CFX 384 Real-time System qRT-PCR machine (Bio-Rad). All primers were designed using PerlPrimer and were purchased from Invitrogen. Primers used are as follows (5′-3′): OTUB1 forward: ACAGAAGATCAAGGACCTCCA, reverse: CAACTCCTTGCTGTCATCCA, FoxO4 forward: TTGGAGAACCTGGAGTGTGACA, reverse: AAGCTTCCAGGCATGACTCAG, PAI-1 forward: AGCTCCTTGTACAGATGCCG, reverse: ACAACAGGAGGAGAAACCCA, CTGF forward: GGAGATTTTGGGAGTACGG, reverse: TACCAATGACAACGCCTCCT, GAPDH forward: TGCACCACCAACTGCTTAGC, reverse: GGCATGGACTGTGGTCATGAG, RPL13A forward: CCTGGAGGAGAAGAGGAAAGAGA, reverse: TTGAGGACCTCTGTGTATTTGTCAA. The primer efficiency was determined and taken into account when evaluating the qRT-PCR data. The data were normalized to the geometrical mean of two housekeeping genes ( GAPDH , RPL13A ). The Pfaffl method [55] was used to analyse the qRT-PCR data in Microsoft Excel. Ubiquitylation/deubiquitylation assays In-cell ubiquitylation/deubiquitylation assays were performed in HEK293 cells by co-transfecting FLAG-SMAD3, HA-ubiquitin and appropriate HA-OTUB1/OTUB1 mutants or NEDD4L constructs. In vitro ubiquitylation/deubiquitylation assays were performed with human recombinant E1, E2 and E3 enzymes, GST-OTUB1 or mutants and SMAD proteins (expressed and purified by DSTT, Axel Knebel or Ubiquigent). For chain cleavage assays, DUBs (30 ng μl −1 ) were incubated in DUB buffer (50 mM Tris–HCl pH 7.5, 5 mM DTT, 100 mM NaCl) with the indicated ubiquitin chains (0.13 μg μl −1 , K48 ub 2–7 , K63 ub 2–7 (Boston Biochem), K48 ub 2 (Axel Knebel)) on an IP shaker for 1 h at 30 °C. Ubiquitylation assays of SMAD2 or FLAG-SMAD2/3/4 (immunoprecipitated from HEK293 cells treated with 50 pM TGFβ for 1 h before lysis) were performed in ubiquitylation assay buffer (50 mM Tris–HCl pH 7.5, 5 mM MgCl2, 2 μM ATP) with His 6 -UBE1 (0.1 μM), UBE2D1 (1 μM or indicated concentrations), His 6 -NEDD4L (1 μM) and ubiquitin (50 μM; Sigma) for 1 h at 30 °C on an IP shaker. The DUBs (30 ng μl −1 or at increasing concentrations (8–60 ng μl −1 )) were added at the start of the ubiquitylation assay (time 0). In vitro DUB assays of in vivo polyubiquitylated FLAG-SMAD2/3/4 (FLAG-SMAD2/3/4 were co-expressed with HA-NEDD4L and HA-ubiquitin in HEK293 cells, treated with 50 pM TGFβ and 10 μM bortezomib for 3 h and FLAG was immunoprecipitated) or in vitro- polyubiquitylated SMAD3 were performed with indicated DUBs in DUB buffer for 1 h at 30 °C on an IP shaker. Proteins were resolved by SDS-PAGE and were immunoblotted. For E2 ubiquitin-loading assays, reactions were performed in 25 μl buffer (50 mM HEPES, 150 mM NaCl, 0.5 mM TCEP) using His 6 -UBE1 (0.5 μg), UBE2D1 (2 μg), FLAG-ubiquitin (2 μg; Sigma), GST-OTUB1 (5.5 μg), His 6 -NEDD4L (1.4 μg), SMAD3 (0.55 μg) and 2 μl Mg-ATP solution (2 mM ATP, 100 mM Mg-acetate). Proteins were mixed on an IP shaker before the addition of ATP for 10 min at 30 °C. After ATP addition, proteins were mixed for a further 10 min at 30 °C before terminating the reaction with 4 × LDS sample buffer. Ten microlitres of each reaction was separated by SDS-PAGE. The gels were stained with Coomassie InstantBlue (Expedeon) and imaged. Cellular migration assay HaCaT cells stably expressing control shRNA or OTUB1 shRNA were seeded to near-confluency into migration inserts (Ibidi) and transfected with FoxO4 or OTUB1 siRNAs , respectively. After 24 h the inserts were removed, the cells were serum starved for 4 h and stimulated with TGFβ (50 pM). Cellular migration was monitored and pictures were taken every 24 h. Statistical analysis All experiments have a minimum of three biological replicates. Luciferase experiments additionally have three and qRT-PCR experiments four technical repeats for each biological repeat. Data are presented as the mean with error bars indicating the s.d. Statistical significance of differences between experimental groups was assessed with Student’s t -test. Differences in means were considered significant if P <0.05. Differences with P <0.05 are annotated as *, P <0.01 are annotated as ** and P <0.001 are annotated as ***. All western blots shown are representative of biological replicates. How to cite this article: Herhaus, L. et al . OTUB1 enhances TGFβ signalling by inhibiting the ubiquitylation and degradation of active SMAD2/3. Nat. Commun. 4:2519 doi: 10.1038/ncomms3519 (2013).